Ag3PO4enables the generation of long-lived radical cations for visible light-driven [2 + 2] and [4 + 2] pericyclic reactions Photocatalytic redox reactions are important for synthesizing fine chemicals from olefins, but the limited lifetime of radical cation intermediates severely restricts semiconductor photocatalysis efficiency. Here, we report that Ag 3 PO 4 can efficiently catalyze intramolecular and intermolecular [2 + 2] and Diels-Alder cycloadditions under visible-light irradiation. The approach is additive-free, catalyst-recyclable. Mechanistic studies indicate that visible-light irradiation on Ag 3 PO 4 generates holes with high oxidation power, which oxidize aromatic alkene adsorbates into radical cations. In photoreduced Ag 3 PO 4 , the conduction band electron ( e CB − ) has low reduction power due to the delocalization among the Ag + -lattices, while the particle surfaces have a strong electrostatic interaction with the radical cations, which considerably stabilize the radical cations against recombination with e CB − . The radical cation on the particle’s surfaces has a lifetime of more than 2 ms, 75 times longer than homogeneous systems. Our findings highlight the effectiveness of inorganic semiconductors for challenging radical cation-mediated synthesis driven by sunlight. Aromatic alkene radical cations, which are one electron (1e)-oxidation intermediates of aromatic alkenes, play important roles in the synthesis of complex functionalized molecules and cyclic moieties, particularly the [2 + 2] and [4 + 2] pericyclic products. To generate and make use of aromatic alkene radical cations, extensive efforts have been devoted for a long time. Compared to single electron oxidants such as Ce 4+ [1] , Fe 3+ [2] , and hypervalent iodine reagents [3] , [4] , photocatalysts (PCs) generate highly oxidizing holes under sunlight irradiation and operate under mild conditions, making photocatalysis a green and sustainable strategy for radical cation-mediated reactions [5] , [6] , [7] , [8] , [9] , [10] , [11] , [12] , [13] , [14] , [15] , [16] . However, the PCs utilized for generating radical cations are primarily homogeneous organic compounds, particularly transition metal-coordination complexes [8] , [9] , [10] , [11] and π-conjugated molecules [12] , [13] , [14] , [15] . Meanwhile, the scope of the approaches is constrained by the short lifetime of radical cations (on a μs scale [17] , [18] , [19] , [20] , [21] , [22] , [23] ). In contrast, inorganic semiconductor PCs (isPCs), such as TiO 2 , CdS, Bi 2 MoO 6 , and Ag 3 PO 4 , have been widely employed for solar light harvesting applications, including water splitting, organic pollutant degradation, and photoelectric conversion [24] . From a practical standpoint, they are generally considered stable, recyclable, inexpensive, and environmentally friendly, making them an ideal choice for use in photosynthesis [25] . However, the efficiency of isPCs in the 1e-oxidative activation of non-polar and non-coordinative C = C moieties on their surfaces is typically low [17] , [20] , [26] , [27] , [28] , [29] , [30] , [31] , [32] , [33] . One obstacle is the short lifetime of holes (fs to ns [34] ), which significantly slows down the 1e-oxidation of the C = C moieties (Fig. 1a ). Moreover, even if some alkene radical cations are slowly generated at the surfaces of a traditional isPC like TiO 2 , they undergo few intermolecular C-C formation reactions [17] . Instead, they are more prone to nucleophilic attack by long-lived photogenerated electrons ( e CB − ), resulting in ineffective 1e-oxidation. These hindrances lead to a diminished quantum yield of light (i.e. reduced reaction rate) and low product yield, regardless of reaction time. Therefore, it is imperative to extend the lifespan of alkene radical cations for affordable and recyclable PCs that can effectively harvest sunlight for pericyclic reactions. However, this remains an ongoing challenge. Fig. 1: The selection of an inorganic semiconductor for photocatalytic pericyclic reactions. a Requirements for using anethole radical cation ( 1a •+ ) in photocatalytic constructing functionalized molecules from anethole ( 1a ). b The band positions of Ag 3 PO 4 and commonly applied photocatalysts. Full size image Among all the available isPCs, Ag 3 PO 4 stands out as one of the few that exhibits an inherent visible-light response [35] . It has been extensively used in visible-light-driven water oxidation [35] , [36] , [37] and organic pollutant degradation [37] , [38] . Compared to other commonly used semiconductors, it produces strong oxidizing holes and weak reducing electrons under visible-light irradiation (+2.9 V and +0.45 V vs . NHE; Fig. 1b ). Moreover, the surfaces of Ag 3 PO 4 are rich in large PO 4 3− anions with high charge density that can strongly electrostatically interact with cationic species such as radical cations. As a result, photo-excited Ag 3 PO 4 may efficiently generate but inefficiently quench radical cations, allowing for the accumulation of radical cations to facilitate radical cation-mediated reactions. In this work, we demonstrate that Ag 3 PO 4 efficiently catalyzes intramolecular and intermolecular [2 + 2] and Diels-Alder cycloadditions under visible light or solar irradiation. The system exhibits remarkable efficiency with respect to substrate scope, product yield, diastereoselectivity, apparent quantum yield (AQY), and scaleup synthesis under solar irradiation. Two critical aspects of the reaction mechanism are validated: (1) the existence of long-lived 1a •+ radical cations on the surfaces of Ag 3 PO 4 that are photo-reduced in situ, (2) the acceleration of rate-limiting step by prolonging the lifetime of 1a •+ . Our discoveries may pave the way for employing highly active organic radical cations and even radical anions in critical pericyclic processes. Transformation of aromatic alkene 1a to anti -cyclobutane 2a Anethole ( 1a ) has been the most studied electron-rich β -substituted styrene in [2 + 2] cycloaddition reactions [3] , [19] , [39] . Therefore, it was selected as the model compound to evaluate the photocatalytic performance of Ag 3 PO 4 (Fig. 2 ). A self-synthesized Ag 3 PO 4 sample composed of nanospheres with a diameter of 230 ± 60 nm was used for the study (Fig. 3a ). The cycloaddition reaction was conducted under an N 2 atmosphere by irradiating a suspension of reactant 1a in hexafluoroisopropanol (HFIP) solvent containing a catalytic quantity of Ag 3 PO 4 (9.0 g L −1 dosage, 0.12 equiv) at 0 °C. No additive was introduced. The conversion of 1a proceeded smoothly, affording anti -cyclobutane 2a as the sole product (see Supplementary Fig. 1 for the time-resolved 1 H NMR spectra and kinetics). After 12 h of reaction, the yield of 2a reached 82%, with a high diastereoselectivity ( d.r . > 19:1). Further irradiation did not affect conversion due to equilibration between 1a and 2a (Supplementary Fig. 2 ), as commonly observed in photocatalyzed radical cation processes [39] , [40] . 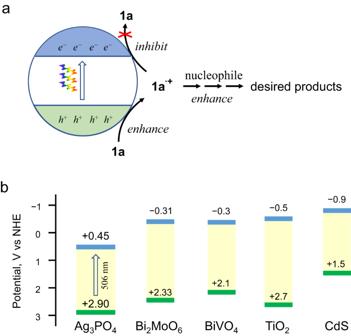Fig. 1: The selection of an inorganic semiconductor for photocatalytic pericyclic reactions. aRequirements for using anethole radical cation (1a•+) in photocatalytic constructing functionalized molecules from anethole (1a).bThe band positions of Ag3PO4and commonly applied photocatalysts. Due to this equilibrium, the 82% yield was also achieved using various Ag 3 PO 4 samples, including a commercially available Ag 3 PO 4 and several self-synthesized faceted Ag 3 PO 4 nanocrystal samples (see Supplementary Table 1 for screening of the experimental conditions). This implies that the catalyst is easily accessible. Fig. 2: The model reaction of 1a. Conditions: 1a , 1 mmol; Ag 3 PO 4 , (27 mg, 0.12 equiv); HFIP, 3.0 mL; LED (425 nm); 1 atm N 2 ; 0 °C; 12 h. Full size image Fig. 3: Characterization of Ag 3 PO 4 and the yields of 2a under various conditions. a An SEM image of Ag 3 PO 4 . b The UV-vis diffuse-reflectance spectrum (smooth blue curve) and the AQY action spectrum (red diamond marks; see Supplementary Information for calculation method) of Ag 3 PO 4 . c The conversion of 1a (green) and yield of 2a (red) during reuse of Ag 3 PO 4 . d The conversion of 1a (green) and yield of 2a (red) by various photocatalysts. The unspecified conditions in panels b – d : 1a , 0.5 mmol; catalyst, 0.12 equiv; HFIP, 1.5 mL; light source, 425 ± 10 nm LED (120 mW cm −2 ); N 2 atmosphere; 0 °C; 12 h. In panel d , a 395 ± 10 nm LED lamp (119 mW cm −2 ) was used for TiO 2 . The reaction time was optimized for each photocatalyst, reaching up to 24 h for TiO 2 . The yields were determined by 1 H NMR using 4-ethoxybenzaldehyde as the internal standard. Full size image The control experiments demonstrated that in the absence of Ag 3 PO 4 or light, no conversion of 1a occurred (Supplementary Table 1 ). Therefore, both light and Ag 3 PO 4 are indispensable for the reaction, excluding the possibility of a thermocatalytic mechanism. Notably, the [2 + 2] cycloaddition reaction requires an inert atmosphere. Under air atmosphere, the conversion of 1a could reach 100%, but 4-methoxybenzaldehyde was the main product (82% yield). The yield of the cycloaddition product 2a was only 13%. This suggests that Ag 3 PO 4 facilitates the selective oxidation of aromatic alkenes, resulting in the formation of the corresponding aromatic aldehydes, when O 2 participates in the reaction process. We also performed the reaction in other solvents like tetrahydrofuran (THF), MeOH, EtOAc, and CF 3 CH 2 OH, but they were not as effective as HFIP. As shown in Fig. 3b , Ag 3 PO 4 can effectively harvest visible light up to 500 nm to initiate the 1a → 2a cycloaddition, which is close to its absorption edge. The AQY values were determined according to the initial 30-min yields. The action spectrum of AQY matches the UV-vis diffuse-reflectance spectrum of Ag 3 PO 4 . The UV-vis absorption spectrum of 1a shows it can only absorb light below 320 nm, and only Ag 3 PO 4 can be excited by the light source (Supplementary Fig. 3 ). Although we were aware that depositing AgNPs on the surfaces of Ag 3 PO 4 could enhance its photo-absorption and charge-separation efficiency [41] , our experiments using AgNPs-loaded samples with different AgNPs’ loadings afforded lower yields than pure Ag 3 PO 4 . Furthermore, as the loading of AgNPs increased, the final yield of 2a decreased (Supplementary Figs. 4 – 6 ). This suggests that AgNPs are not the photocatalyst and can inhibit the activity of Ag 3 PO 4 . In all, it can be concluded that Ag 3 PO 4 is the true photocatalyst, and all 2a is the product of Ag 3 PO 4 photocatalysis. Silver salt-based photocatalysts often suffer from photocorrosion [42] , [43] , [44] , [45] . However, in the current system, the 0.12 equiv of initially added Ag 3 PO 4 successfully worked five consecutive photocatalytic cycles with only a slight decrease in efficiency (Fig. 3c ), resulting in a turnover number of 13. Photo-corrosion of Ag 3 PO 4 was observed, as evidenced by its significant darkening after five cycles. The TEM image indicates the formation of numerous AgNPs on the surfaces of Ag 3 PO 4 (Supplementary Fig. 7 ). Nevertheless, regeneration of the recycled sample was achieved through a simple immersion in 6.7 mM Na 2 HPO 4 aqueous solution and the addition of a drop of 30% H 2 O 2 [46] . Within minutes, color, microscopic morphology, and photocatalytic performance were fully restored (Supplementary Fig. 7 ). As shown in Fig. 3d , when the other silver salts, such as AgCl, AgBr, and AgI, were used, the conversion of 1a and the selectivity of 2a were significantly lower than that of Ag 3 PO 4 . Both commercially available and self-synthesized AgCl, AgBr, and AgI decomposed rapidly upon irradiation (see Supplementary Fig. 8 for characterization). In comparison to the widely studied heterogeneous photocatalysts [47] , including graphitic carbon nitride (g-C 3 N 4 ), Bi 2 MoO 6 , and TiO 2 , the performance of Ag 3 PO 4 is superior. For example, the reaction rate was notably low over TiO 2 even under UV. Furthermore, electron accumulation caused TiO 2 to exhibit a blue hue and ultimately became completely inert once conversion reached 18% (Supplementary Fig. 9 ). When TiO 2 was used under air atmosphere, the accumulated electrons can be efficiently quenched by O 2 . However, in this case the yield of 2a was less than 10% due to the over-oxidization of 1a to 4-methoxybenzaldehyde (67%). 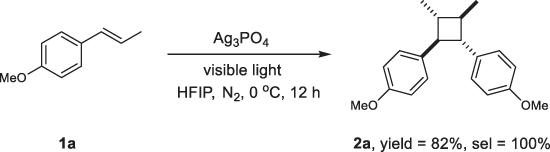Fig. 2: The model reaction of 1a. Conditions:1a, 1 mmol; Ag3PO4, (27 mg, 0.12 equiv); HFIP, 3.0 mL; LED (425 nm); 1 atm N2; 0 °C; 12 h. Supplementary Table 2 shows that Ag 3 PO 4 performs comparably to state-of-the-art PCs and single-electron oxidants such as Ru(bpm) 3 (BArF) 2 [39] , PhI(OAc) 2 3 and Fe(ClO 4 ) 3 in the 1a → 2a cycloaddition [19] . Therefore, Ag 3 PO 4 is highly applicable for [2 + 2] cyclobutanation reactions. Ag 3 PO 4 /visible light system for pericyclic reactions Given the success of the [2 + 2] homo-cycloaddition of 1a , we sought to explore whether the Ag 3 PO 4 /visible light system could serve as a versatile tool for achieving various pericyclic reactions. Our initial focus was on investigating the scope of the intermolecular dimerization reaction. As shown in Fig. 4 , a diverse range of electron-rich aromatic alkenes with varying substituents underwent smooth reaction, affording the corresponding symmetrical cyclobutanes in moderate to good yields and excellent diastereoselectivity ( 2a - 2h , yield ranges 42%-83%, d.r . > 19:1). Electronic density of the aromatic ring and steric hindrance at the β -site exert a noticeable influence on the reaction outcome ( 2b vs. 2c, 2a vs . 2d - 2f ). However, this catalytic system exhibits high tolerance toward steric hindrance at the benzene ring ( 2a vs . 2f - 2h ). 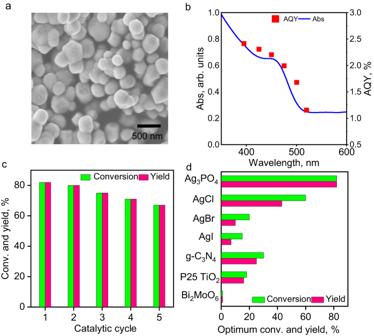Fig. 3: Characterization of Ag3PO4and the yields of 2a under various conditions. aAn SEM image of Ag3PO4.bThe UV-vis diffuse-reflectance spectrum (smooth blue curve) and the AQY action spectrum (red diamond marks; seeSupplementary Informationfor calculation method) of Ag3PO4.cThe conversion of1a(green) and yield of2a(red) during reuse of Ag3PO4.dThe conversion of1a(green) and yield of2a(red) by various photocatalysts. The unspecified conditions in panelsb–d:1a, 0.5 mmol; catalyst, 0.12 equiv; HFIP, 1.5 mL; light source, 425 ± 10 nm LED (120 mW cm−2); N2atmosphere; 0 °C; 12 h. In paneld, a 395 ± 10 nm LED lamp (119 mW cm−2) was used for TiO2. The reaction time was optimized for each photocatalyst, reaching up to 24 h for TiO2. The yields were determined by1H NMR using 4-ethoxybenzaldehyde as the internal standard. Notably, NO 2 -, OH-, and COOH-substituted aromatic alkenes were challenging substrates for other [2 + 2] cycloaddition catalytic systems [48] , as well as the current Ag 3 PO 4 system (Supplementary Table 3 ). Finally, we achieved a 70% isolated yield of magnosalin ( 2h ), a valuable natural product. We then used the system to synthesize unsymmetric cyclobutanes and were pleased to discover that a variety of aromatic alkenes, including unsubstituted aromatic alkene ( 4a ) and substituted aromatic alkenes with electron-donating groups (EDGs; 4b, 4d, 4i ) and electron-withdrawing groups (EWGs; 4c, 4e, 4f, 4g, 4h ) at both ortho-, meta- and para-sites of the benzene rings, could be employed as model reaction counterparts using 1a . 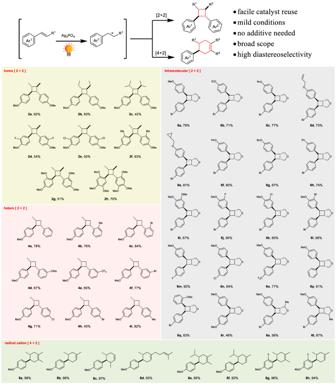Fig. 4: Scope of the Ag3PO4photocatalysis in the radical cation pericyclic reactions. aConditions for homo [2 + 2] reactions: substrate, 1.0 mmol; Ag3PO4, 27 mg (0.12 equiv); 12–18 h.bConditions for hetero [2 + 2] reactions:1a, 0.5 mmol; the counterpart, 1.0 mmol; Ag3PO4, 44 mg (0.20 equiv); 12 h.cConditions for intramolecular [2 + 2] reactions: substrate, 0.3 mmol; Ag3PO4, 12 mg (0.10 equiv); 12 h.dConditions for [4 + 2] reactions: aromatic alkene, 1.0 mmol; diene, 2.0 mmol; Ag3PO4, 32 mg (0.08 equiv); 8 h. The corresponding intermolecular [2 + 2] products ( 2a − 2h and 4a − 4i ) were obtained in high yields and high regioselectivity (head-to-head; see Supplementary Table 4 for 1 H NMR analysis). The sole byproduct resulting from these crossed reactions is the homo-cycloaddition product, e.g., 2a . 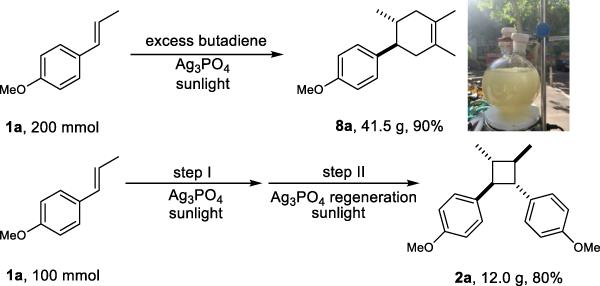Fig. 5: Scaleup synthesis using sunlight. Detailed reaction conditions were described in theSupplementary Information. However, because the crossed reactions are much faster than the homo-cycloaddition (see Supplementary Fig. 10 for a comparison of the rates), introducing 1a via a syringe pump would inhibit the homo [2 + 2] reaction. Next, we explored the feasibility of intramolecular [2 + 2] cycloaddition, an efficient approach for synthesizing fused heterocycles [6] . Strikingly, all tested bis(styrene)s afforded good to excellent yields of the desired cyclobutanes ( 6a - 6t ). The intramolecular [2 + 2] cycloadditions exhibit a broad tolerance toward EDGs, EWGs, and the steric hindrance at both the benzene ring and the β -site. The Diels-Alder reaction is considered one of the essential C-C bond-forming reactions in synthetic organic chemistry. Recent studies have shown that photocatalytic methods are effective in the radical-cation-mediated cycloadditions of electron-rich olefins and dienes [32] , [49] , [50] , [51] , [52] , which are challenging substrates for conventional thermal processes. In this study, we found that even with a reduced Ag 3 PO 4 loading of 0.08 equiv, the Ag 3 PO 4 /visible light system was still capable of facilitating Diels-Alder cycloadditions involving the radical cations. Moreover, the 0.08 equiv of Ag 3 PO 4 was successfully reused for five consecutive runs without any noticeable decrease in performance (Supplementary Figure 11 ). Based on the substituted aromatic alkenes, the yields achieved in all tested reactions are near unity ( 8a - 8h ). The products 8b, 8c, 8d, 8f, and 8h were isolated in high regioselectivity without isomers. This can be attributed to the large steric hindrance of the butadiene side chain (see Supplementary Table 4 for 1 H NMR analysis). Fig. 4: Scope of the Ag 3 PO 4 photocatalysis in the radical cation pericyclic reactions. a Conditions for homo [2 + 2] reactions: substrate, 1.0 mmol; Ag 3 PO 4 , 27 mg (0.12 equiv); 12–18 h. b Conditions for hetero [2 + 2] reactions: 1a , 0.5 mmol; the counterpart, 1.0 mmol; Ag 3 PO 4 , 44 mg (0.20 equiv); 12 h. c Conditions for intramolecular [2 + 2] reactions: substrate, 0.3 mmol; Ag 3 PO 4 , 12 mg (0.10 equiv); 12 h. d Conditions for [4 + 2] reactions: aromatic alkene, 1.0 mmol; diene, 2.0 mmol; Ag 3 PO 4 , 32 mg (0.08 equiv); 8 h. Full size image The remarkable diastereoselectivity of the reactions is noteworthy. Specifically, nearly all intermolecular [2 + 2] products are anti; intramolecular [2 + 2] products are predominately syn, and nearly all Diels-Alder reactions yield anti-products. Scale synthesis of [2 + 2] and [4 + 2] reactions To investigate the synthetic potential of the Ag 3 PO 4 /visible light system, we performed large-scale [2 + 2] and [4 + 2] reactions under natural sunlight irradiation by placing the reaction flasks on a windowsill at outdoor temperatures (1–10 °C). The sunlight intensity ranged from 15−23 mW cm −2 . Interestingly, 41.5 g of the [4 + 2] cycloaddition product 8a was obtained almost quantitatively in a one-pot reaction after only six hours of irradiation (Fig. 5 ). After being filtered through diatomite, the Ag 3 PO 4 solid was removed, resulting in nearly pure 8a (41.5 g), which confirms the method’s flexibility and ease of use. The intermolecular [2 + 2] homo-cycloaddition of 1a yielded a 60% yield of 2a (100% selectivity) before Ag 3 PO 4 (0.05 equiv) became deactivated. However, upon reintroduction of regenerated Ag 3 PO 4 into the catalytic system, a final yield of 80% of 2a was achieved (Fig. 5 ). The use of a 425 nm LED lamp achieved yields of 8a that are comparable to that achieved by sunlight (Supplementary Table 1 ). Hence, the Ag 3 PO 4 /visible light system could facilitate actual industrial production considering the advances in LED technology. Fig. 5: Scaleup synthesis using sunlight. Detailed reaction conditions were described in the Supplementary Information . Full size image Supplementary Tables 5 – 7 demonstrate the superior performance of the Ag 3 PO 4 /visible light system compared to the state-of-art reports in [2 + 2] and Diels-Alder cycloadditions. The current system boasts one of the highest efficiencies in heterogeneous systems, with broad light absorption. It is capable of realizing intramolecular and intermolecular [2 + 2] cycloadditions and Diels-Alder reactions. Mechanism study and DFT simulations Laser flash photolysis (LFP) was performed to detect the transient species involved in the photocatalytic 1a → 2a cycloaddition. The LFP transient absorption spectra of the 1a /Ag 3 PO 4 /HFIP suspension were obtained in transmission mode. The representative spectra are depicted in Fig. 6a . The two distinct, intense peaks centered at ca. 387 and 605 nm precisely match the spectra of 1a •+ generated by photolysis of homogeneous solutions of 1a /H 2 O-MeCN at 266 nm [53] and 1a /MeCN at 308 nm [54] , respectively, as reported in previous studies. 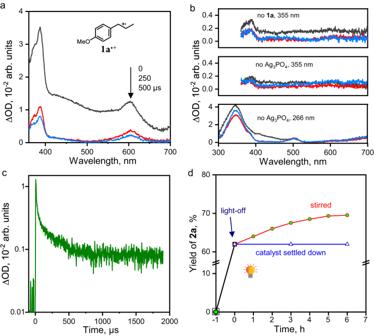Fig. 6: Detection of the transient species. aTransient absorption spectra of1a•+obtained at various times after a 10-ns 355-nm pulse irradiation of the1a/Ag3PO4/HFIP system at room temperature under an air atmosphere. Before LFP, the suspension was ultrasonicated for 30 min to enhance the dispersion of Ag3PO4in HFIP.bThe transient absorption spectra obtained without1aor Ag3PO4: black,t= 0; red, 250 μs; blue, 500 μs.cThe decay kinetics of1a•+after 355-nm pulse irradiation.dThe kinetics of2aformation in the light on-off experiment. Figure 6b demonstrates that the absence of 1a or Ag 3 PO 4 resulted in no signal from a 355-nm laser pulse, indicating the indispensability of both 1a and Ag 3 PO 4 for the formation of 1a •+ . Hence, the LFP spectra confirm that photogenerated h + of Ag 3 PO 4 facilitates the 1e-oxidation of 1a to afford 1a •+ . Fig. 6: Detection of the transient species. a Transient absorption spectra of 1a •+ obtained at various times after a 10-ns 355-nm pulse irradiation of the 1a /Ag 3 PO 4 /HFIP system at room temperature under an air atmosphere. Before LFP, the suspension was ultrasonicated for 30 min to enhance the dispersion of Ag 3 PO 4 in HFIP. b The transient absorption spectra obtained without 1a or Ag 3 PO 4 : black, t = 0; red, 250 μs; blue, 500 μs. c The decay kinetics of 1a •+ after 355-nm pulse irradiation. d The kinetics of 2a formation in the light on-off experiment. Full size image The concentration of a transient species, which is determined by both formation rate and lifetime, is essential for detecting it via LFP. Hence, the observation of 1a •+ in the 1a /Ag 3 PO 4 /HFIP system suggests that 1a •+ forms rapidly and has a long life, allowing for its accumulation due to its formation far exceeding decay. Recall Fig. 6a , the sample initially exhibited strong background absorption, which significantly decreased after 250 μs due to the sedimentation of Ag 3 PO 4 particles. The spectra at 250 and 500 μs showed similar level of background absorption, indicating that sedimentation was minor during this period. Based on this understanding, we measured the decay kinetics of 1a •+ in the 1a /Ag 3 PO 4 /HFIP suspension at λ = 600 nm. Figure 6c demonstrates that the signal intensity decayed significantly before 500 μs, which could be mostly attributable to the sedimentation mentioned above of Ag 3 PO 4 . Afterward, the signal intensity remained nearly constant until 1900 μs. This must not be attributed to the continuous generation of 1a •+ by the photogenerated holes of Ag 3 PO 4 after LFP, because it is well-known that the photogenerated holes in semiconductors are transient species. Instead, this indicates that the lifetime of 1a •+ in the 1a /Ag 3 PO 4 /HFIP system is more than 1900 μs. We conducted light-on-off experiments to investigate the lifetime of 1a •+ in the 1a /Ag 3 PO 4 /HFIP system. The reaction vial was either left stirring in the dark after turning off the light or centrifuged to settle down the Ag 3 PO 4 before being left in the dark. In the former situation, over the next six hours, there was a gradual increase of ca. 8% in yield of 2a (Fig. 6d ). This is distinct from the homogeneous systems, where the 1a → 2a cycloaddition practically ceased upon light-off [55] . In the dark reaction without agitation, the yield of 2a remained unchanged after Ag 3 PO 4 settled down (Fig. 6d ). It indicates that the long-lived 1a •+ radical cations must remain adsorbed on the surfaces of the reduced Ag 3 PO 4 (denoted as (Ag 3 PO 4 ) n − , where n is the number of e CB − per NP). When all the Ag 3 PO 4 particles settled down, the 1a molecules in solution could not reach 1a •+ , and thus the cycloaddition ceased. This verifies that the signals originate from 1a •+ adsorbed on the Ag 3 PO 4 surfaces rather than in the solution bulk. Further, it confirms that the radical cation-mediated [2 + 2] pericyclic reaction occurs on the surfaces of Ag 3 PO 4 rather than in the solution. It was reported that the decay rate constant [53] , [56] of 1a •+ is 4 × 10 4 s −1 in aerated MeCN, corresponding to a very short lifetime of 25 μs [54] . This is likely why the 1a → 2a cycloaddition stopped nearly instantly upon light-off in homogeneous systems [22] , [55] . To probe the lifetime of 1a •+ in neat HFIP, we used a 266-nm laser pulse to excite a 1a /HFIP solution. However, the system produced signals from unknown species and the absorption peaks of 1a •+ at ca. 387 and 605 nm were not detected. This may suggest that the lifetime of 1a •+ in HFIP is too short, resulting in a 1a •+ concentration below the detection limit. We also used a 355-nm laser pulse to excite the 1a /TiO 2 /HFIP system, which produced a 16% yield of 2a , indicating that photo-excited TiO 2 NPs generated 1a •+ . However, the transient spectrum of 1a •+ was not detected by LFP (Supplementary Fig. 12 ), implying that its lifetime in the system is also very short. We found that the adsorption of reactant 1a and desorption of product 2a are crucial in the reaction. 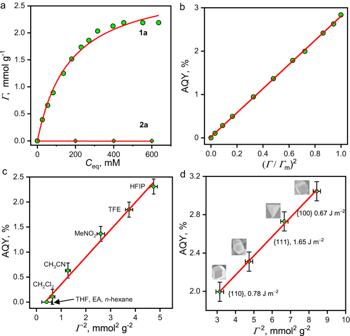Fig. 7: Dependence of AQY on adsorption. aThe adsorption isotherm of1aand2aon spherical Ag3PO4.b–dThe AQY values of the1a→2acycloaddition reaction as functions of (Г/Гm)2orГ2. The scattered points represent the experimental values, and the red lines are the curve fit or linear fits. Abbreviations for panelc: THF tetrahydrofuran, EA ethyl acetate, TFE trifluoroethanol. The SEM images, facets, and surface energies of Ag3PO4NPs are indicated in panel d. The error bars in panels (c) and(d) associated with AQY represent the standard error of three sets of unique measurements. Figure 7a shows that the adsorption of 1a on the (100)-facet-rich spherical Ag 3 PO 4 (as the representative example) can fit well to the Langmuir type-I isotherm (Eq. 1 ), 
    =_m·K·C_eq/(1+K·C_eq)
 (1) where Г is the adsorbed amount at the adsorption/desorption equilibrium concentration C eq . The Langmuir coefficient K and the capacity of adsorption Г m are calculated to be 5.8 ± 0.6 M −1 and 2.9 ± 0.1 mmol g −1 , respectively. In contrast, the adsorption of 2a on Ag 3 PO 4 surfaces is barely detectable, indicating very weak adsorption of 2a . Fig. 7: Dependence of AQY on adsorption. a The adsorption isotherm of 1a and 2a on spherical Ag 3 PO 4 . b – d The AQY values of the 1a → 2a cycloaddition reaction as functions of ( Г / Г m ) 2 or Г 2 . The scattered points represent the experimental values, and the red lines are the curve fit or linear fits. Abbreviations for panel c : THF tetrahydrofuran, EA ethyl acetate, TFE trifluoroethanol. The SEM images, facets, and surface energies of Ag 3 PO 4 NPs are indicated in panel d. The error bars in panels ( c ) and( d ) associated with AQY represent the standard error of three sets of unique measurements. Full size image At low 1a concentrations, the AQY values increase dramatically with the initially added concentration of 1a but then approach a plateau (Supplementary Fig. 13 ). This differs from a typical homogeneous bimolecular reaction, which is second order depending on the substrate concentration. Instead, the AQY values are well linearly correlated with the square of the fractional coverage of 1a, Ɵ (Eq. 2 ), 
    AQY=k(/_m)^2=k θ^2
 (2) where k denotes the slope of the plot (Fig. 7b ). This kinetic equation corroborates that the conversion of 1a through photocatalysis occurs on the Ag 3 PO 4 surface. The rate-limiting step (RLS) of the formation of 2a involves two molecular species of 1a adsorbed on the surface. We also observe a significant solvent effect in the performance of Ag 3 PO 4 in the 1a → 2a cycloaddition reaction (Fig. 7c ). Ag 3 PO 4 did not perform well in EtOAc, n -hexane or CH 2 Cl 2 , but performed better in CH 3 CN, MeNO 2 , and TFE, and performed best in HFIP. Surprisingly, Eq. 2 applies to the results from different solvents. Thus, solvents influence the AQY by modulating the 1a distribution between the bulk solution and Ag 3 PO 4 surfaces. It has been reported that the facets of photocatalysts substantially influence their activities, especially in the case of Ag 3 PO 4 [36] , [37] , [57] , [58] . For the 1a → 2a cycloaddition reaction, we used the spherical, rhombic dodecahedral, cubic, and tetrahedral NPs of Ag 3 PO 4 , which are rich in {100}, {110}, {100}, and {111} facets, respectively [36] . Figure 7d displays distinct AQYs on different facets and Eq. 2 is applicable to the results from various Ag 3 PO 4 facets. Overall, Fig. 7 indicates that the photocatalytic cycloaddition reaction on Ag 3 PO 4 surfaces follows the Langmuir-Hinshelwood mechanism for a bimolecular reaction. It also implies that the interaction between 1a and Ag 3 PO 4 surfaces is vital in the success of Ag 3 PO 4 in the photocatalytic [2 + 2] cycloadditions. We conducted DFT simulations to determine the mechanism of interfacial interactions between 1a (and 2a ) and the Ag 3 PO 4 surfaces. Given the substantial dimensions of the Ag 3 PO 4 particles and the comparable sizes of 1a or 2a molecules to only a few phosphate anions, it is reasonable to regard the surface of Ag 3 PO 4 particles as an infinitely expansive plane for adsorbing 1a and 2a . As the (100) facet is the lowest-energy facet of Ag 3 PO 4 crystals [36] , [37] , [58] and the primary surface of spherical Ag 3 PO 4 , we selected the PO 4 3− -terminated and the Ag + -terminated (100) facets to calculate the optimal adsorption configurations (see Supplementary Figs. 14 – 15 for details of results). 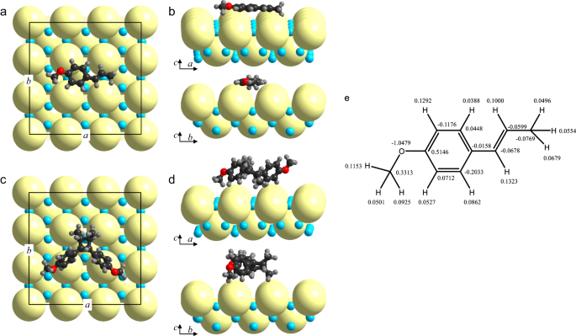Fig. 8: Configurations of adsorption and Bader charge. a–dThe lowest-energy configurations of1aand2amolecules on the 2 × 2 region of the PO43−-terminated (100) facet of Ag3PO4.aandcare the top views.banddare the side views. The labelsaandbdenote the cell axes. The pale-yellow spheres represent PO43−(r= 2.38 Å), and the cyan spheres represent Ag+(r= 0.67 Å).1aand2amolecules are drawn to scale.eThe atomic Bader charges of adsorbed1a. Figure 8 displays the lowest-energy configurations of 1a and 2a molecules on the PO 4 3− -terminated (100) facet. It should be noted that the size of PO 4 3− is much larger than that of Ag + (2.38 Å vs. 0.67 Å), but comparable to molecule 1a in size. Molecule 1a lies parallel to the facet, with its long axis aligned with the a -axis of the crystal lattice, and the CH = CH moiety positioned close to the O 2− ions of PO 4 3− . In this configuration, each 1a molecule intimately contacts four PO 4 3− anions, maximizing the interfacial interaction between 1a and the Ag 3 PO 4 surface. The strong interaction is consistent with the previously discussed adsorption of 1a to the Ag 3 PO 4 surfaces. This adsorption mode should be beneficial for the 1e-oxidation of the CH = CH moiety upon photo-excitation of Ag 3 PO 4 since photogenerated holes are localized at O of PO 4 3− [59] . The energy required for adsorption of each 1a molecule from the vacuum is −2.10 eV (Fig. 8a, b ). In contrast, the calculated energies for 1a adsorption onto PO 4 3− -terminated (100) facet along the b -axis and that onto the Ag + -terminated (100) facet along both the a - and b -axis, are substantially smaller at −1.67, −1.54, and −1.54 eV, respectively (Supplementary Fig. 14 ). These lower adsorption energies can be attributed to the greater spacing between the adjacent PO 4 3− anions on these facets, which weakens the contact between 1a and PO 4 3− . However, due to the large steric effects of the 2a molecule, each 2a has an optimum adsorption energy of −1.56 eV when adsorbed on the PO 4 3− -terminated (100) facet (Fig. 8c, d ). The above calculations reveal a large adsorption energy difference between two 1a and one 2a , i.e. +2.64 eV on the PO 4 3− -terminated Ag 3 PO 4 (100) facet in a vacuum. The much weaker adsorption of 2a suggests that the 1a → 2a cycloaddition on the Ag 3 PO 4 surfaces benefits from the easier removal of product 2a . Fig. 8: Configurations of adsorption and Bader charge. a – d The lowest-energy configurations of 1a and 2a molecules on the 2 × 2 region of the PO 4 3− -terminated (100) facet of Ag 3 PO 4 . a and c are the top views. b and d are the side views. The labels a and b denote the cell axes. The pale-yellow spheres represent PO 4 3− ( r = 2.38 Å), and the cyan spheres represent Ag + ( r = 0.67 Å). 1a and 2a molecules are drawn to scale. e The atomic Bader charges of adsorbed 1a . Full size image The atomic Bader charges shown in Fig. 8e indicate that the electron density of 1a changes upon adsorption. The overall Bader charge of adsorbed 1a is 0.34e, indicating a transfer of 0.34e from 1a to the Ag 3 PO 4 surfaces during adsorption. The two H-atoms in the CH = CH moiety have enormous Bader charges, namely, 0.1323e and 0.1e, respectively. This, combined with the very negative Bader charge of the CH 3 O moiety ( − 0.4587e), strongly suggests that polarization occurs in molecule 1a and that its CH = CH group is activated upon adsorption. The high Bader charge also means that the CH = CH group is the most readily oxidized site in 1a . 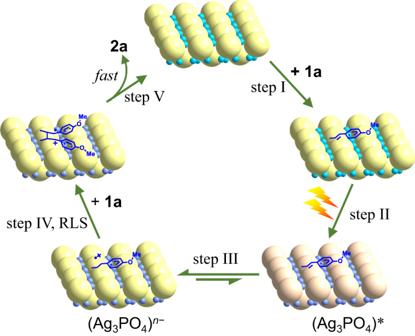Fig. 9: A plausible mechanism. (Ag3PO4)* denotes a photo-excited Ag3PO4NP with manyeCB−andh+. The purple-blue spheres are used to show that in (Ag3PO4)* and (Ag3PO4)n−, theeCB−is shared by silver cations, resulting in a fraction charge ofδ+ (0 <δ< 1) on each cation. Figure 9 illustrates a plausible mechanism for Ag 3 PO 4 triggering the [2 + 2] cycloaddition of 1a under visible-light irradiation. Initially, Ag 3 PO 4 adsorbs 1a molecules on its surface via PO 4 3− anions (step I). Then, upon excitation, Ag 3 PO 4 generates many e CB − in the conduction band and h + in the valance band (step II). Due to the fact that the conduction band bottom is mainly composed of hybridized Ag 5s5p orbitals [35] , the reduction power of the electrons in the conduction band of Ag 3 PO 4 is low ( E CB = +0.45 V vs. NHE [35] , [41] , [60] , [61] ). The unreactive e CB − remains in the form of (Ag δ+ ) m − , which means it is shared by many Ag + ions. The observed AgNP formation substantiates that e CB − transfers to Ag + ions. The valance band top of Ag 3 PO 4 mainly comprises hybridized O 2p and Ag 4d orbitals. The h + in the valence band has strong oxidation power ( E VB = +2.90 V vs. NHE [35] , [41] , [60] , [61] ) and is able to gain an electron from the CH = CH group of 1a to yield 1a •+ (step III). The 1e-oxidation of 1a results in the photocatalytically reduced NP with numerous e CB − . The 1a •+ species strongly adsorbs on the surfaces of (Ag 3 PO 4 ) n − . In this case, the electrostatic interaction between 1a •+ and (Ag 3 PO 4 ) n − NP surfaces is analogous to the interactions in homogeneous solutions described by Yoon et al. for 1a •+ with a tetraarylborate anion [18] , Ishihara et al. for 1a •+ with FeCl 4 − [19] , [20] , [21] , and List et al. for 1a •+ with an imidodiphosphorimidate counteranion [22] . Fig. 9: A plausible mechanism. (Ag 3 PO 4 )* denotes a photo-excited Ag 3 PO 4 NP with many e CB − and h + . The purple-blue spheres are used to show that in (Ag 3 PO 4 )* and (Ag 3 PO 4 ) n − , the e CB − is shared by silver cations, resulting in a fraction charge of δ + (0 < δ < 1) on each cation. Full size image The adsorbed 1a •+ is stabilized by electrostatic interaction with the (Ag 3 PO 4 ) n − surfaces. The low possibility recombination between 1a •+ and e CB − shared by multiple Ag + cations, (Ag δ+ ) m − , is evidenced by the observation of AgNP formation. As a result, the lifetime of 1a •+ is dramatically prolonged to > 2 ms, which is over 75 times longer than in a homogeneous solution (μs level [54] ). The long lifetime of 1a •+ benefits the nucleophilic attack by another adsorbed 1a molecule, allowing the reaction of 1a + 1a •+ → 2a •+ in step IV to proceed (the RLS; see Supplementary Information for analysis). The final step (step V) is the ring closure reaction of 2a •+ . The potential of 2a •+ / 2a is approximately +1.5 V vs . NHE, much higher than the E CB of Ag 3 PO 4 . Thermodynamically, the transfer of an electron from the reduced Ag 3 PO 4 to 2a •+ is an exothermic reaction. Step V may also occur through a radical chain mechanism [22] . Considering the potential of 1a •+ / 1a , which is approximately +1.3 V vs . NHE, the ring closure of 2a •+ by e CB − exhibits a much larger driving force than that by the radical chain process. The ability to generate the long-lived radical cation 1a •+ distinguishes (Ag 3 PO 4 ) n − from a traditional photocatalytically reduced TiO 2 NP. On the illuminated TiO 2 NP, the lifetime of 1a •+ was too short to detect, and the conversion was only 18% (Fig. 3d ). Okada et al. used a substantial excess of TiO 2 (e.g., > 6 equiv) to minimize the accumulated electron per NP and extra LiClO 4 (1.0 M) to stabilize the radical cations [18] , [22] , [23] , [25] , [26] , [27] . In contrast, Ag 3 PO 4 photocatalysis can harvest the visible spectrum of sunlight and achieve a high yield of the desired product without any additives. Ag 3 PO 4 is a powerful photocatalyst for homo, crossed, intramolecular [2 + 2], and Diels-Alder [4 + 2] pericyclic reactions under visible-light irradiation. The catalytic process is mild, straightforward, affordable, additive-free, scalable under sunlight irradiation, and allows for easy product separation and catalyst reuse. It has a broad substrate scope and produces a wide range of desired products in modest to excellent yields. Our study reveals the potential of this photocatalytic process for fine chemical production. We have demonstrated that the rate-limiting step is the reaction between the reactant and its 1e-oxidation intermediate, a radical cation. The lifetime of anethole radical cation ( 1a •+ ) on the Ag 3 PO 4 surfaces exceeds 2 ms, which is over 75 times longer than that in the homogeneous solutions, thus effectively promoting the rate-limiting step. The long lifetime of 1a •+ is attributed to the appropriate band structure of Ag 3 PO 4 and the strong electrostatic interaction between 1a •+ and the (Ag 3 PO 4 ) n − NP surfaces, which should be a general and essential mechanism for promoting chemical processes mediated by radical cations on heterogeneous surfaces. This may inspire ideas for more challenging radical cation/anion-mediated solar synthesis using inorganic semiconductor photocatalysts. General procedure for the photocatalytic reactions The reactions were carried out in 10-mL Pyrex vials. Olefin and Ag 3 PO 4 were dispersed in a solvent in the vial, which was then purged for 10 min with high-purity N 2 (99.999%). The vial was immersed in a mixture of ice and water to maintain the reaction temperature. The reaction suspension was stirred in the dark for 30 min to achieve adsorption-desorption equilibrium. The mixture was then exposed to the lamp from the side. To monitor the reaction progress, a syringe was used to withdraw 10 μL of the solution for analysis by thin-layer chromatography (TLC). After the reaction, the suspension was centrifuged to separate the solid catalyst from the solution. The residue is purified with column chromatography to afford the desired pure products. Details for the homo-dimerization of aromatic alkenes To a solution of aromatic alkene 1 (1.0 mmol) in 3.0 mL of HFIP, Ag 3 PO 4 (27 mg, 0.12 equiv) was added in one portion. The remaining steps are the same as the general procedure. Details for the cross-dimerization of aromatic alkenes To a solution of aromatic alkene 3 (1.0 mmol, 2.0 equiv) in 2.0 mL of HFIP was added Ag 3 PO 4 (44 mg, 0.20 equiv). Then, the reaction mixture was degassed by purging with high-purity nitrogen for 10 min. An ice bath was used to maintain the reaction temperature. The mixture was stirred in the dark at 0 °C for half an hour to achieve adsorption-desorption equilibrium. The photocatalytic reaction was then initiated by irradiating the dispersion from the side with the LED lamps. During the reaction, a solution of 1 (0.5 mmol) in 2.0 mL HFIP was added using a syringe pump (at a rate of 4.0 mL/h). The remaining steps are the same as the general procedure. Details for the intramolecular [2 + 2] reactions To a solution of aromatic alkene 5 (0.3 mmol) in 2.0 mL of HFIP, Ag 3 PO 4 (12 mg, 0.10 equiv) was added in one portion. The remaining steps are the same as the general procedure. Details for the Diels–Alder cycloadditions To a solution of the diene 7 (2.0 mmol, 2.0 equiv) in 2.0 mL of HFIP was added Ag 3 PO 4 (32 mg, 0.08 equiv). Then, the reaction mixture was degassed by purging with high-purity nitrogen for 10 min. An ice bath was used to maintain the reaction temperature. The mixture was then stirred in the dark at 0 °C for half an hour to achieve adsorption-desorption equilibrium. The photocatalytic reaction was initiated by irradiating the dispersion from the side with an LED lamp. During the reaction, a solution of 1 (1.0 mmol) in 2.0 mL of HFIP was added using a syringe pump (at a rate of 4.0 mL/h). The remaining steps are the same as the general procedure.